The p53–PUMA axis suppresses iPSC generation Mechanisms underlying the reprogramming process of induced pluripotent stem cells remain poorly defined. Like tumorigenesis, generation of induced pluripotent stem cells was shown to be suppressed by the Trp53 (p53) pathway, at least in part via p21 Cdkn1a (p21)-mediated cell cycle arrest. Here we examine the role of PUMA, a pro-apoptotic mediator of p53, during somatic reprogramming in comparison to p21 in the p53 pathway. Using mouse strains deficient in these molecules, we demonstrate that PUMA is an independent mediator of the negative effect of p53 on induced pluripotent stem cell induction. PUMA deficiency leads to a better survival rate associated with reduced DNA damage and fewer chromosomal aberrations in induced pluripotent stem cells, whereas loss of p21 or p53 results in an opposite outcome. Given these new findings, PUMA may serve as a distinct and more desirable target in the p53 pathway for induced pluripotent stem cell generation, thereby having important implications for potential therapeutic applications of induced pluripotent stem cells. The reprogramming of differentiated cells into induced pluripotent stem cells (iPSCs) by introduction of four defined transcription factors (Oct4, Sox2, Klf4 and Myc) has rapidly become an intensively investigated area in stem cell research given its great promise in regenerative medicine [1] , [2] , [3] , [4] . The full therapeutic potential of the iPSC technology depends on a thorough understanding of the biological mechanisms underlying the reprogramming process. Both genetic and epigenetic programs may contribute to the process of iPSC reprogramming [3] , [5] , [6] . The reprogramming toward iPSC has been elegantly modelled as a stochastic process that can be accelerated by both cell-division-rate-dependent and cell-division-rate-independent manners [7] . These two models were experimentally achieved by inhibiting the p53–p21 axis and increasing the expression of Nanog, respectively. However, the cell death parameter was neglected in both models. In fact, a closer examination by single-cell tracking revealed a higher fraction of the aberrant iPSC colonies when p53 was knocked down during the reprogramming [8] , thereby suggesting other important checkpoints on cell death and potential genomic instability yet to be defined during the reprogramming. Genomic instability is a controversial topic in iPSC generation. On the one hand, studies using a genome-wide scanning approach have documented higher genomic instability in iPSCs compared to that in embryonic stem cells (ESCs) at least within a certain spectrum of cell lines, reinforcing the importance of further evaluating the key molecular circuit for the genomic stability of established iPSC lines [9] , [10] , [11] , [12] . On the other hand, some recent data indicated that reprogramming is a mutation-free process [13] , [14] and that iPSCs and ESCs are equally unstable [15] . p53 is the best known ‘guardian’ of the genome [16] , [17] . In response to stress, p53 activates multiple cellular processes, including cell cycle arrest, apoptosis and DNA repair [18] . p53 halts cell cycle progression via induction of CDK inhibitors, such as p21 Cdkn1a (p21), which enables DNA repair or renders cells susceptible to senescence. In parallel, p53 triggers cell death via the activation of apoptotic proteins, such as p53-upregulated mediator of apoptosis (PUMA), a BH-3-only pro-apoptotic protein in the Bcl-2 family [19] , [20] . Activation of the p53 pathway suppressed iPSC generation and in contrast, abrogation of p53 increased the efficiency of induction [21] , [22] , [23] , [24] , [25] , [26] , [27] . Similarly, knocking down p21 by RNA interference also increased the efficiency of iPSC induction [21] . In spite of the documented importance of the p53–p21 axis during iPSC reprogramming [22] , the specific role of the p53–PUMA axis has not been defined during the reprogramming. PUMA is a potent mediator of apoptosis due to its broad interactions with other Bcl-2 family members under a variety of stress conditions [28] . Previous studies, including ours, have shown that loss of PUMA protects hematopoietic stem cells and intestinal stem cells from high-dose ionizing radiation by diminishing apoptosis in response to p53 activation [29] , [30] , [31] , [32] , [33] . Importantly, loss of PUMA does not seem not to increase carcinogenesis in general [29] , [30] , [31] , [32] , [34] , [35] . In the current study, we examine iPSC generation from murine cells that are deficient in PUMA, p21 or p53 in order to dissect the unique effect of PUMA in comparison with p21 and p53 during somatic reprogramming. We found that although loss of both PUMA and p21 abrogates the inhibitory effect of p53 on iPSC colony formation, cellular consequences of the loss of PUMA or p21 differ significantly. PUMA depletion leads to a better survival rate associated with reduced DNA damage and fewer chromosomal aberrations in iPSCs in comparison to the loss of p21 or p53. Our results demonstrate that PUMA is a limiting factor for the reprogramming of iPSCs through induction of apoptosis and expectedly genomic instability. Inhibitory effects of PUMA and p21 or p53 on iPSC induction To explore the potential role of PUMA in the reprogramming process, we first analyzed the expression of PUMA, along with p53 and p21, at the protein level using western analysis during the induction of iPSCs from mouse embryonic fibroblasts (MEFs). The results showed that PUMA protein level was barely detectable and significantly lower than those of p53 and p21 before transduction. However, it was upregulated at day 1 after retroviral transduction of the four transcription factors (4F) and continued to increase throughout the period of 12 days in culture ( Fig. 1a ). Like PUMA, protein levels of both p53 and p21 were also increased over the course. We subsequently focused on the quantification of the efficiencies of iPSC colony formation from the MEF cells that were deficient in p53 ( p53 −/− ), p21 ( p21 −/− ) or PUMA ( PUMA −/− ) in comparison with the wild-type (WT) MEF cells. Briefly, the same number of MEFs of each genotype were seeded and then transduced with the 4F retrovirus cocktail for the induction of iPSC generation [36] . Comparable transduction efficiencies (40–65%) with the retroviruses were achieved between different groups. The induced cell colonies were seen around day 12 after transduction with 4F ( Supplementary Fig. S1 ). The colonies were initially screened at day 14 by examining alkaline phosphatase (AP) activity ( Fig. 1b ), a method that was previously used to indicate reprogramming potential [21] , [25] , [27] . Strikingly, the absence of PUMA, p53 or p21 in MEFs all enhanced AP + colony formation to a similar degree by more than 10-fold compared with that of WT MEFs. Furthermore, to better indicate the primitiveness of the reprogrammed cells, we enumerated the colonies that stained positive for two primitive stem cell markers, SSEA1 and Nanog, at day 21 after the transduction with 4F ( Supplementary Fig. S2 ). The yield of the colonies co-expressing SSEA1 and Nanog was consistent with the result by AP staining, further demonstrating the enhanced induction of iPSCs in the absence of p53, p21 or PUMA ( Fig. 1d ). Especially, PUMA −/− group produced the highest number of SSEA + /Nanog + colonies. Conversely, overexpression of PUMA, p21 or p53 cDNA in WT or knockout MEF cells significantly suppressed the generation of SSEA1 and Nanog double-positive cells ( Supplementary Fig. S3 ). 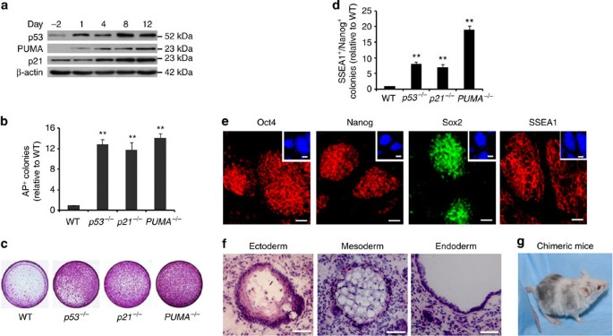Figure 1: PUMA reduces iPSC reprogramming efficiency at a comparable level to p53 or p21. (a) Western blot analysis of PUMA, p53 and p21 expression during iPSC generation. Cells were collected and lysed at the indicated time points after transduction with the four transcription factors (Oct4, Sox2, Klf4 and C-myc). β-actin was used as a control. (b) AP-positive colony numbers inp53−/−,p21−/−andPUMA−/−iPSCs relative to that of WT iPSCs at day 14 after transduction. (c) Representative dishes of AP staining of iPSC colonies derived from MEFs in different genotypes. (d) SSEA1 and Nanog double-positive colonies inp53−/−,p21−/−andPUMA−/−iPSCs relative to that of WT iPSCs at day 21 after transduction. (e) Immunostaining of iPSCs using antibodies against Oct4, Nanog, Sox2 or SSEA1. Representative results fromPUMA−/−iPSCs were shown. Bars: 50 μm. Insets: DAPI staining of the nuclei (reduced scale to 1/13). (f) Teratomas derived fromPUMA−/−iPSCs. Hematoxylin and Eosin stainings of ectoderm, mesoderm and endoderm layers. Bars: 50 μm. (g) Chimeric mouse generated fromPUMA−/−iPSCs. Error bars inbandd, s.e.m. Statistical significance was tested using the one-way ANOVA with Newman–Keuls post-test (bandd). **P<0.01. Results ina,frepresent three independent experiments with similar results. Figure 1: PUMA reduces iPSC reprogramming efficiency at a comparable level to p53 or p21. ( a ) Western blot analysis of PUMA, p53 and p21 expression during iPSC generation. Cells were collected and lysed at the indicated time points after transduction with the four transcription factors (Oct4, Sox2, Klf4 and C-myc). β-actin was used as a control. ( b ) AP-positive colony numbers in p53 −/− , p21 −/− and PUMA −/− iPSCs relative to that of WT iPSCs at day 14 after transduction. ( c ) Representative dishes of AP staining of iPSC colonies derived from MEFs in different genotypes. ( d ) SSEA1 and Nanog double-positive colonies in p53 −/− , p21 −/− and PUMA −/− iPSCs relative to that of WT iPSCs at day 21 after transduction. ( e ) Immunostaining of iPSCs using antibodies against Oct4, Nanog, Sox2 or SSEA1. Representative results from PUMA −/− iPSCs were shown. Bars: 50 μm. Insets: DAPI staining of the nuclei (reduced scale to 1/13). ( f ) Teratomas derived from PUMA −/− iPSCs. Hematoxylin and Eosin stainings of ectoderm, mesoderm and endoderm layers. Bars: 50 μm. ( g ) Chimeric mouse generated from PUMA −/− iPSCs. Error bars in b and d , s.e.m. Statistical significance was tested using the one-way ANOVA with Newman–Keuls post-test ( b and d ). ** P <0.01. Results in a , f represent three independent experiments with similar results. Full size image Establishment of iPSC lines in the absence of PUMA To verify whether the derived iPSCs had acquired a typical ESC-like phenotype, we generated induced cell lines from emerging colonies with WT, PUMA −/− , p53 −/− , p21 −/− or PUMA −/− / p21 −/− genotype, and focused on the PUMA −/− genotype because it has not been evaluated in the setting of reprogramming experiments before. We examined the expression of multiple markers for pluripotency, including Oct4, Nanog, Sox2 and SSEA1 in all iPSC colonies ( Fig. 1e ). The co-expression of these primitive markers correlated with the quality of iPSC colonies as judged by the morphology ( Supplementary Fig. S4 ). Among all the genotypes, PUMA −/− iPSCs exhibited the healthiest morphology as compared to other groups. To confirm the pluripotency of PUMA −/− iPSCs in vivo , we injected WT or PUMA −/− iPSCs into NSG immunodeficient mice to assess the formation of teratomas. Both WT and PUMA −/− iPSC groups produced teratomas that could differentiate into all three germ layers ( Fig. 1f ). Importantly, we were able to produce chimeric pups by injecting PUMA −/− iPSCs, but not p53 −/− or p21 −/− induced cells (~60–100 embryos injections/induced cell line) into blastocysts ( Fig. 1g , Supplementary Table S1 ), confirming the pluripotency of PUMA −/− -induced cells. Reprogramming of p53 −/− , PUMA −/− or p21 −/− MEFs with three transcription factors (3F) without Myc produced similar results ( Supplementary Fig. S5b ). A similar result was also obtained from the reprogramming of c-Kit + -enriched bone marrow hematopoietic stem and progenitor cells to iPSCs. Moreover, a gene-dose effect of iPSC generation, which led to an intermediate phenotype between WT and KO, was observed in all of the heterozygous MEFs with either 4F or 3F ( Supplementary Fig. S5 ). Knockdown of PUMA by shRNAs during human iPSC generation significantly enhanced the efficiencies of iPSC colony formation ( Supplementary Fig. S6 ). Taken together, these data clearly demonstrated that in addition to p53 and p21, PUMA is a potent and non-redundant blocker for iPSC generation in the p53 pathway. The findings also seem to indicate that PUMA −/− iPSCs are more competent than p53 −/− or p21 −/− iPSCs. Independent roles of PUMA and p21 during iPSC reprogramming We next sought to further quantify the effects of PUMA, p21 and p53 during somatic reprogramming using complementation experiments. We first ectopically expressed p53 WT or a nonfunctional mutant p53 S58A in p21 −/− or PUMA −/− MEF cells and then induced iPSC formation. As shown in Fig. 2a , overexpression of WT p53 inhibited iPSC colony formation in p21 −/− or PUMA −/− MEF cells, whereas overexpression of p53 S58A did not. Conversely, when overexpressed in p53 −/− MEF cells, either PUMA or p21 was able to partially restore the suppression of p53 on iPSC colony formation ( Fig. 2c ), further suggesting that p53 suppresses iPSC induction through both p21 and PUMA. Moreover, as p53 activity is negatively regulated by MDM2 (refs 21 , 37 ), we physiologically activated p53 protein, by using MDM2 inhibitor Nutlin-3a (refs 21 , 37 ), in MEFs of different genotypes. As expected, Nutlin-3a largely inhibited iPSC formation in WT MEFs ( Fig. 2d ), but not in p53 −/− MEFs ( Fig. 2e ). Consistent with the result ( Fig. 2a ), Nutlin-3a partially inhibited iPSC generation in both p21 −/− and PUMA −/− MEFs ( Fig. 2f ), further supporting that both PUMA and p21 are required for p53-mediated suppression of iPSC induction. Our results also reinforce the notion that inhibiting cell proliferation can block reprogramming. 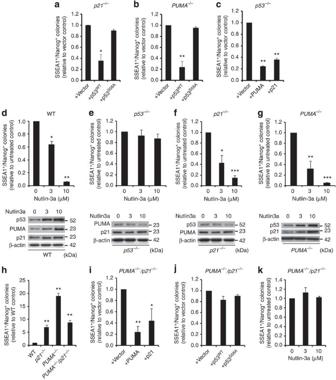Figure 2: PUMA and p21 independently mediate p53-induced inhibition of iPSC generation. (a,b) Overexpression of p53 inp21−/−orPUMA−/−MEFs.p21−/−(a) orPUMA−/−(b) MEFs were separately transduced with retroviruses encoding p53WT, mutant p53S58Aor an empty vector along with 4F. (c) Overexpression of p21 and PUMA inp53−/−MEFs.p53−/−MEFs were transduced with retroviruses encoding PUMA, p21 or an empty vector along with 4F. (d–g) Inhibition of iPSC generation by activation of p53. The WT (d),p53−/−(e),p21−/−(f) andPUMA−/−(g) MEFs were transduced with 4F. After transduction, cultures of each genotype of MEFs were separated equally into three groups and treated with Nutlin-3a (0, 3 or 10 μM). The SSEA1+/Nanog+colonies from all the groups were counted at day 21 after transduction and the numbers were normalized to that of the untreated in each group. Western blots show the expression of PUMA, p53 and p21 in various genotype MEFs at day 4 of reprogramming treated with different concentrations of Nutlin-3a. (h) iPSC reprogramming efficiency in singlePUMAnull,p21null or double null compared with that in wild type. Various MEFs were transduced with retroviruses encoding 4F. (i,j) Effects of ectopic expression of PUMA, p21 and p53 on iPSC generation inPUMA−/−/p21−/−MEFs.PUMA−/−/p21−/−MEFs were transduced with retroviruses carrying PUMA (i), p21 (i), p53WT(j), mutant p53S58A(j) or an empty vector along with 4F. (k) Activation of p53 during the iPSC generation ofPUMA−/−/p21−/−MEFs.PUMA−/−/p21−/−MEFs were infected with retroviruses encoding 4F and treated with Nutlin-3a (0, 3 and 10 μM) after transduction. The numbers of colonies were normalized to that of WT, the vector control or the untreated, respectively. Error bars ina–k, s.e.m. Statistical significance was tested using the one-way ANOVA with Newman–Keuls post-test (a–k). *P<0.05, **P<0.01, ***P<0.001. Results ina–krepresent three independent experiments with similar results. Figure 2: PUMA and p21 independently mediate p53-induced inhibition of iPSC generation. ( a , b ) Overexpression of p53 in p21 −/− or PUMA −/− MEFs. p21 −/− ( a ) or PUMA −/− ( b ) MEFs were separately transduced with retroviruses encoding p53 WT , mutant p53 S58A or an empty vector along with 4F. ( c ) Overexpression of p21 and PUMA in p53 −/− MEFs. p53 −/− MEFs were transduced with retroviruses encoding PUMA, p21 or an empty vector along with 4F. ( d – g ) Inhibition of iPSC generation by activation of p53. The WT ( d ), p53 −/− ( e ), p21 −/− ( f ) and PUMA −/− ( g ) MEFs were transduced with 4F. After transduction, cultures of each genotype of MEFs were separated equally into three groups and treated with Nutlin-3a (0, 3 or 10 μM). The SSEA1 + /Nanog + colonies from all the groups were counted at day 21 after transduction and the numbers were normalized to that of the untreated in each group. Western blots show the expression of PUMA, p53 and p21 in various genotype MEFs at day 4 of reprogramming treated with different concentrations of Nutlin-3a. ( h ) iPSC reprogramming efficiency in single PUMA null, p21 null or double null compared with that in wild type. Various MEFs were transduced with retroviruses encoding 4F. ( i , j ) Effects of ectopic expression of PUMA, p21 and p53 on iPSC generation in PUMA −/− /p21 −/− MEFs. PUMA −/− /p21 −/− MEFs were transduced with retroviruses carrying PUMA ( i ), p21 ( i ), p53 WT ( j ), mutant p53 S58A ( j ) or an empty vector along with 4F. ( k ) Activation of p53 during the iPSC generation of PUMA −/− /p21 −/− MEFs. PUMA −/− /p21 −/− MEFs were infected with retroviruses encoding 4F and treated with Nutlin-3a (0, 3 and 10 μM) after transduction. The numbers of colonies were normalized to that of WT, the vector control or the untreated, respectively. Error bars in a – k , s.e.m. Statistical significance was tested using the one-way ANOVA with Newman–Keuls post-test ( a – k ). * P <0.05, ** P <0.01, *** P <0.001. Results in a – k represent three independent experiments with similar results. Full size image These findings indicated that both PUMA and p21 have independent and non-overlapping roles in p53-mediated inhibition of iPSC reprogramming. However, it is unclear whether PUMA and p21 are the major mediators of p53-induced suppression of iPSC colony formation. To address this question, we generated PUMA −/− /p21 −/− double-knockout mice and then obtained PUMA −/− /p21 −/− MEFs for iPSC generation. As expected, deletion of both PUMA and p21 markedly enhanced the formation of iPSC colonies in a degree similar to p53 deletion ( Fig. 2h ). Ectopic expression of either PUMA or p21 in PUMA −/− /p21 −/− MEFs partially restored the inhibition of p53 on iPSC colony formation ( Fig. 2i ), similar to the effect of overexpressed PUMA or p21 in p53 −/− MEFs ( Fig. 2c ). In contrast, overexpression of p53 by retroviral delivery ( Fig. 2j ) or activation of p53 by Nutlin-3a ( Fig. 2k ) in PUMA −/− /p21 −/− MEFs failed to inhibit the formation of SSEA1 + /Nanog + colonies, indicating that p53 suppression on iPSC induction is largely, if not entirely, dependent on p21 and PUMA. Effects of PUMA and p21 on iPS reprogramming efficiency PUMA is a specific mediator of mitochondria mediated-apoptosis [28] , [34] , [35] . We therefore examined the effect of apoptosis on the reprogramming efficiency by analyzing the expression of Annexin V in the transduced MEFs at different time points. The number of apoptotic cells increased during the later stages (8 days after transduction) of reprogramming in WT and p21 −/− ( Fig. 3a–c ). In contrast, apoptosis in the PUMA −/− or p53 −/− groups did not increase throughout the reprogramming ( Fig. 3a–c ). The TUNEL assay further confirmed these findings ( Fig. 3d ). These results support that p53 suppresses iPSC generation, in part, through triggering PUMA-dependent apoptosis. Notably, the apoptotic rate was the highest in p21 −/− cells, whereas it was lower in the PUMA −/− /p21 −/− , and similar in PUMA −/− and p53 −/− groups, indicating that PUMA null suppresses increased apoptosis induced by p21 null during the reprogramming process. This result was also consistent with the poor quality of the p21 −/− iPSCs as reflected by the morphology ( Supplementary Fig. S4 ). 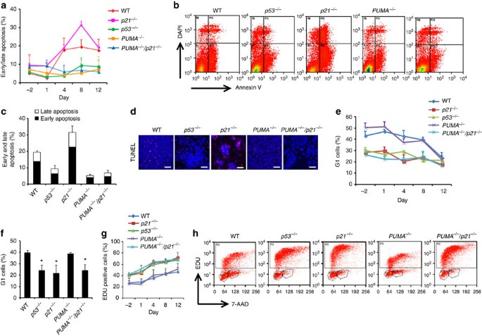Figure 3: Distinct effects on apoptosis and cell cycle during iPSC reprogramming. (a) Flow cytometry (FACS) analysis of apoptosis in various genotype MEFs at different time points during iPSC reprogramming. WT,PUMA−/−,p21−/−,p53−/−andPUMA−/−/p21−/−MEFs were transduced with retroviruses encoding 4F, respectively. Cells were collected at different time points, stained with Annexin V and DAPI and analyzed by FACS. WT MEFs without viral transduction were used as negative controls (n=3 in each group). Early apoptosis, Annexin V+/DAPI-cells; late apoptosis, Annexin+/DAPI+cells. (b) Representative profiles of FACS analysis of apoptosis at day 8 after retroviral transduction. (c) FACS analysis of apoptosis at day 8 after infection. (d) Representative images ofin situdetection of apoptotic cells by TUNEL assay ( × 20 objective lens). MEFs were cultured on glass coverslips in the wells of 24-well plates. At day 8 after retroviral transduction, cells were fixed with 2% paraformaldehyde and stained with TUNEL. Bars, 50 μm. (e) and (f) FACS analysis of cell cycle by EDU and 7-AAD staining at different time points during reprogramming (e) and at day 8 after tranduction G1-phase cells were negative for EDU staining and positive for 7AAD staining (intensity at 64 as shown in `h'). (g) Proliferation measured by EDU staining in different genotype MEFs at different time points during iPSC reprogramming. (h) Representative profiles of FACS analysis of cell cycle at day 8 after retroviral transduction. Error bars ina,cande–g, s.e.m. Statistical significance was tested using the one-way ANOVA with Newman–Keuls post-test (a,c,e–g). *P<0.05. Results ina–hrepresent three independent experiments with similar results. Figure 3: Distinct effects on apoptosis and cell cycle during iPSC reprogramming. ( a ) Flow cytometry (FACS) analysis of apoptosis in various genotype MEFs at different time points during iPSC reprogramming. WT, PUMA −/− , p21 −/− , p53 −/− and PUMA −/− /p21 −/− MEFs were transduced with retroviruses encoding 4F, respectively. Cells were collected at different time points, stained with Annexin V and DAPI and analyzed by FACS. WT MEFs without viral transduction were used as negative controls ( n =3 in each group). Early apoptosis, Annexin V + /DAPI - cells; late apoptosis, Annexin + /DAPI + cells. ( b ) Representative profiles of FACS analysis of apoptosis at day 8 after retroviral transduction. ( c ) FACS analysis of apoptosis at day 8 after infection. ( d ) Representative images of in situ detection of apoptotic cells by TUNEL assay ( × 20 objective lens). MEFs were cultured on glass coverslips in the wells of 24-well plates. At day 8 after retroviral transduction, cells were fixed with 2% paraformaldehyde and stained with TUNEL. Bars, 50 μm. ( e ) and ( f ) FACS analysis of cell cycle by EDU and 7-AAD staining at different time points during reprogramming ( e ) and at day 8 after tranduction G1-phase cells were negative for EDU staining and positive for 7AAD staining (intensity at 64 as shown in `h'). ( g ) Proliferation measured by EDU staining in different genotype MEFs at different time points during iPSC reprogramming. ( h ) Representative profiles of FACS analysis of cell cycle at day 8 after retroviral transduction. Error bars in a , c and e – g , s.e.m. Statistical significance was tested using the one-way ANOVA with Newman–Keuls post-test ( a , c , e – g ). * P <0.05. Results in a – h represent three independent experiments with similar results. Full size image Conversely, we examined cell cycle progression of the reprogramming cells during the time course. As shown in Fig. 3e , following transduction with 4F, the percentage of G1-phase cells of all genotypes decreased and the cell proliferation rates increased. However, at the early stage (day 4) and middle stage (day 8) after transduction, the percentages of G1 stage cells in the groups with p53 −/− , p21 −/− and PUMA −/− /p21 −/− genotypes were significantly lower than that with WT and PUMA −/− genotypes, which correlated with increased cell proliferation rates measured by EDU incorporation ( Fig. 3g ). Notably, compared with the WT culture, no difference was found in the cell cycle progression and proliferation rate between PUMA −/− and WT cultures. Therefore, PUMA does not have a measurable impact on cell cycle progression during the reprogramming. Marion et al. [25] reported that knockdown of p53 or p21 increases DNA damage during iPSC reprogramming. In contrast, deletion of PUMA has been associated with reduced DNA damage in hematopoietic stem cells [31] . To further gain insights into the DNA damage response and genomic maintenance of the iPSCs generated in the absence of these two key regulators of p53 pathway, we examined the double-strand DNA breaks by an antibody against γ-H2AX in the transduced MEF cells at day 4 and the iPSC colonies at days 12 after transduction ( Fig. 4a–c ). Consistent with the previous report [25] , γ-H2AX staining increased significantly in the emerging p53 −/− or p21 −/− iPSC colonies mainly at day 12, compared to WT colonies. In contrast, γ-H2AX staining decreased in the PUMA −/− cells, while it increased in PUMA −/− /p21 −/− iPSC colonies. These results indicate that p21, but not PUMA has a dominant role in suppressing double-strand breaks during iPSC reprogramming. As a result, decreased DNA damage or more efficient DNA repair in the absence of PUMA may attribute to enhanced p21 activity, as suggested by previous studies [31] , [38] . 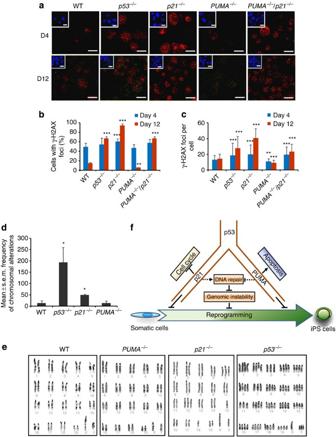Figure 4: The DNA damage and chromosomes instability inPUMA−/−iPSCs are less than those inp21−/−orp53−/−iPSCs. (a) Analysis of double-strand DNA breaks by γ-H2AX foci staining in induced cells with various genotype at day 4 and day 12 after retroviral transduction, respectively. Insets: DAPI staining of the nuclei. Bars, 20 μm. (b) Percentage of cells with γ-H2AX foci. Two hundred induced cells per genotype were analyzed. (c) γ-H2AX foci numbers per induced cell with different genotype in cells with at least three foci. One hundred cells were analyzed per genotype. Error bars inbandc, s.e.m. Results inbandcrepresent three independent experiments with similar results. *P<0.5, **P<0.01 and ***P<0.001. (d) The karyotypic alterations in three clones each from three independent iPSCs at passage 5 derived from three passage 3 MEF cell lines per genotype were quantified. Graphic illustration of the number of chromosomal alterations (numerical gains, losses and structural alterations) in the iPSCs. Error bars, s.e.m. Statistical significance was tested using the one-way ANOVA with Newman–Keuls post-test (b–d). *P<0.5. (e) Karyotypes from 20 metaphase cells from three sets of each three cell lines per type of iPSCs were analyzed under the microscope or after digital imaging and karyotyping. Images shown were taken with × 100 oil objective and represent three independent experiments with similar results. (f) A model of the distinct role of the p53 pathway and key mediators in iPSC generation. Figure 4: The DNA damage and chromosomes instability in PUMA −/− iPSCs are less than those in p21 −/− or p53 −/− iPSCs. ( a ) Analysis of double-strand DNA breaks by γ-H2AX foci staining in induced cells with various genotype at day 4 and day 12 after retroviral transduction, respectively. Insets: DAPI staining of the nuclei. Bars, 20 μm. ( b ) Percentage of cells with γ-H2AX foci. Two hundred induced cells per genotype were analyzed. ( c ) γ-H2AX foci numbers per induced cell with different genotype in cells with at least three foci. One hundred cells were analyzed per genotype. Error bars in b and c , s.e.m. Results in b and c represent three independent experiments with similar results. * P <0.5, ** P <0.01 and *** P <0.001. ( d ) The karyotypic alterations in three clones each from three independent iPSCs at passage 5 derived from three passage 3 MEF cell lines per genotype were quantified. Graphic illustration of the number of chromosomal alterations (numerical gains, losses and structural alterations) in the iPSCs. Error bars, s.e.m. Statistical significance was tested using the one-way ANOVA with Newman–Keuls post-test ( b – d ). * P <0.5. ( e ) Karyotypes from 20 metaphase cells from three sets of each three cell lines per type of iPSCs were analyzed under the microscope or after digital imaging and karyotyping. Images shown were taken with × 100 oil objective and represent three independent experiments with similar results. ( f ) A model of the distinct role of the p53 pathway and key mediators in iPSC generation. Full size image Impact of PUMA and p21 or p53 on chromosome instability Using a genome-wide scanning approach, three research groups recently found higher genomic instability in iPSC in comparison to ESC [9] , [10] , [11] , [12] . Given the different impacts of these genes on iPSC generation and cellular parameters as shown above, we finally examined the consequences of the deletion of these genes on chromosomal instability in the established iPSC lines. We quantified the chromosomal alterations in three clones each from three independent iPSCs at passage 5 derived from three passage 3 MEF cell lines per genotype. Chromosomal alterations, including chromosomal gains, losses, structural abnormalities and ploidy changes were observed and quantified in all four genotypes of the iPSCs and the corresponding MEFs ( Fig. 4d and Supplementary Tables S2–S7 ). Consistent with previous reports [39] , ploidy alterations were expected in the p53 −/− MEFs and iPSCs. The p21 −/− and p53 −/− iPSCs had significantly more chromosomal alterations in comparison to the WT and PUMA −/− iPSCs and the corresponding MEFs ( Fig. 4d ). PUMA −/− and WT iPSCs did not differ from each other. The reduced chromosomal aberrations in p21 −/− compared to p53 −/− iPSCs might be due to increased apoptosis. Some of the observed chromosomal alterations were clonal, but not associated with reprogramming. For example, cytogenetic analysis revealed trisomy 5 in three of nine p21 −/− iPSCs and one of nine PUMA −/− iPSC, but not in p21 −/− sister cell cultures. Trisomy 5 was reported to confer a growth advantage in cell culture as does its human ortholog chromosome 7 (ref. 40 ). We also evaluated anaphase and interphase bridges [41] in various genotype iPSCs at reprogramming day 12 and in their corresponding MEFs ( Supplementary Fig. S7 and Supplementary Table S8 ). Except in p53 null iPSCs, no difference in interphase and anaphase bridges was found among the iPSCs and MEFs. Overall, the chromosomal instability studies suggest that the chromosomal alterations observed in the iPSCs arose largely during the reprogramming process, although some alterations seemed to have been inherited from the original MEFs. In summary, while targeting specific molecular circuitry may enhance our ability to increase the success of iPSC generation, genomic instability should be minimized while self-renewal and pluripotency are reestablished [42] . Overlapping mechanisms between reprogramming and oncogenesis exemplified by the p53 pathway represent a major challenge for the therapeutic use of iPSC technology [24] . The goal of the present study was to gain a better understanding of the specific, yet distinct roles of two major factors downstream of p53 during iPSC reprogramming to identify a more suitable molecular target and potentially improve the technology for human iPSC generation. Given the comparable levels of iPSC reprogramming, preservation of cell survival is accompanied by reduced DNA damage, fewer chromosomal alterations (as demonstrated in our current study), as well as less direct association with tumorigenesis in the absence of PUMA [29] , [30] , [31] , [32] , PUMA may serve as a more desirable target for iPSC generation than other molecules in the p53 pathway ( Fig. 4f ). This conclusion is also echoed by previous studies showing strong resistance to radiation or DNA damage-induced apoptosis without increased incidences of malignancies in the absence of PUMA [29] , [30] , [31] , [32] , [43] . In contrast, our recent study demonstrated that in the absence of another BH-3-only protein, Bid did not confer a survival advantage on stem cells [44] . Moreover, overexpression of Bcl-2 only moderately increased the reprogramming efficiencies (1.8-fold) compared with the vector control. These studies further suggest the uniqueness of targeting PUMA for iPSC generation, as intact cell cycle checkpoints and repair mechanisms, mediated at least in part by p21, might effectively suppress genomic instability induced by a high rate of proliferation required during reprogramming and cellular transformation when apoptosis is compromised [45] . Admittedly, cautions should be also taken as other studies showed that loss of PUMA accelerates Myc -driven tumorigenesis [46] or DSS-driven colon cancer [43] , [47] , [48] . Therefore, strategies for transiently blocking PUMA expression or its protein activity are needed to avoid potential risks associated with long-term PUMA knockdown for therapeutic purposes. Mice PUMA −/− mice were gifts from Dr Gerard P. Zambetti at the St Jude Children’s Research Hospital, Memphis, TN. WT, p21 −/− , p53 −/− mice and NOD/SCID/Gamma (NSG) mice were purchased from The Jackson Laboratory. All of these mouse strains had been crossed to generate a pure C57BL/6J background. PUMA −/− and p21 −/− mice were intercrossed to generate PUMA +/− /p21 +/−- double heterozygous mice and then mated with p21 −/− mice to generate PUMA +/− /p21 −/− littermates. PUMA +/− /p21 −/− littermates were interbred for successive generations to obtain PUMA −/− /p21 −/− double-KO mice. The NOD/SCID/IL-2 receptorγunit deficient (NSG) mice were purchased from The Jackson Laboratory. All mouse strains were maintained in the pathogen-free animal facility of the University of Pittsburgh Cancer Institute. The Institutional Animal Care and Use Committee at the University of Pittsburgh approved all procedures and animal experiments. Cell culture conditions Primary MEFs were obtained from 13.5-day embryos of the indicated genotypes based on the protocol from Wicell (Madison, WI, USA) and cultured in standard DMEM medium containing 10% FBS (Hyclone, Logan, UT). Murine ES and iPSCs were cultured in ‘ES culture medium’ composed of Knock-Out DMEM (Invitrogen, Carlsbad, CA) supplemented with ES cell qualified FBS (15%, Stem Cell Technologies, Vancouver, BC, Canada), LIF (1,000 U ml −1 ), non-essential amino acids, glutamine, and β-mercaptoethanol. Bone marrow c-Kit + cells were harvested from femurs of mice, enriched by CD117-beads (Miltenyi, Auburn, CA), and cultured in standard BIT9500 (Stem Cell Technologies, Vancouver, BC, Canada) containing 10% FBS supplemented with murine SCF, Flt-3 and TPO factors before transduction. Generation of retroviruses The retroviral constructs, pMXs-Klf4, pMXs-Sox2, pMXs-Oct4, pMIG-Bcl-2, pMXs-Myc (4F), mouse p53, as well as a mutated form of mouse p53 (p53 S58A ) were purchased from Addgene (Cambridge, MA). The cDNA of mouse p21 was also purchased from Addgene. The cDNA of mouse PUMA was purchased from Open Biosystems. They were individually cloned into pMXs-GFP retroviral vectors. pMXs-GFP was a gift from Dr Russel O. Pieper of the University of California San Francisco. Retroviral constructs pMXs-hKlf4, pMXs-hSox2, pMXs-hOct4, pMXs-hc-Myc (4F) were purchased from Addgene. hPUMA shRNAs were purchased from Open Biosystems (Lafayette, CO). To produce retroviruses, the indicated plasmids (10 ug per 100 mm dishes) were transfected into Platinum-E retroviral packaging cells (Cell Biolabs, San Diego, CA) using Lipofectamine 2000 (Invitrogen, Carlsbad, CA). Retroviral supernatant was collected 48 and 72 h after transfection and stored at −80 °C. Generation of mouse iPSCs Second-passage MEFs of indicated genotype were seeded in 100-mm diameter dishes (5 × 10 5 cells per dish) pre-coated with 0.1% gelatin (Sigma, St Louis, MO) in DMEM with 10% FBS medium. They were transduced twice in the next 2 days at 24-h intervals with the retroviral supernatant as indicated. At the end of the 48 h transduction period, the culture medium was switched to ES culture medium and changed daily. For the Nutlin-3a experiments, cells were treated once they were transferred to ES culture medium. After 10–12 days in culture, colonies with ES-cell-like morphology became visible. At day 14, the colonies were either scored after alkaline phosphatase staining or picked for further expansion on irradiated feeder fibroblasts using standard ES culture methods. Further, the numbers of SSEA1 and Nanog double-positive colonies were counted on day 21 to score the full reprogramming efficiency. Reprogramming efficiency For quantification of iPSC generation efficiency, retroviral transduction was measured in parallel transductions containing all the retroviruses used for reprogramming plus a GFP retrovirus (pMXs-GFP) (equal volumes of each retrovirus were used during the transduction). The efficiency of transduction was measured by fluorescence-activated cell sorting (FACS) analysis at the day after the medium was switched to ES culture medium. The total numbers of iPSC colonies were counted after staining plates for alkaline phosphatase activity (AP detection kit, Millipore, Billerica, MA). The full reprogramming efficiency was assessed by SSEA1 and Nanog staining. Briefly, 500,000 cells per 100-mm dish were seeded after retroviral transduction. The numbers of SSEA1 and Nanog double-positive colonies were counted on day 21. The percentage of SSEA1 and Nanog double-positive colonies over all the transduced MEFs was determined. The efficiency of reprogramming was also calculated as the relative change compared to that of control. We have used three independent MEF isolates (from distinct foetuses) per genotype for AP staining and another three independent MEF isolates per genotype for SSEA1 and Nanog assays. Generation of human iPSCs Human fibroblasts (ATCC, Manassas, VA, USA) were seeded at 8 × 10 5 cells per 100 mm dish 1 day before transduction. The virus-containing supernatants were filtered through a 0.45-mm pore-size filter and supplemented with 4 mg ml −1 polybrene generated by plat_E cells. Equal amounts of supernatants containing each of the four retroviruses were mixed, transferred to the fibroblast dish, and incubated overnight. Then the PUMA shRNA virus (Open Biosystems) was individually transduced to human fibroblast for one time. At the sixth day after transduction, fibroblasts were harvested by trypsinization and replated at 5 × 10 5 cells per 100 mm dish on a feeder layer. Next day, the medium was replaced with Primate ES cell medium supplemented with 4 ng ml −1 bFGF. The medium was changed every other day. Thirty days after transduction, the colonies were picked up and transferred into a new plate. AP staining and counting were performed. Teratoma formation 2 × 10 6 cells from the indicated mouse induced cell line were injected subcutaneously into NOD/SCID mice. Teratomas were surgically removed after 4 weeks. Tissues were snap-frozen, embedded in tissue-tek with OCT compound, and stored at −80 °C. The samples were sectioned at a thickness of 5 μm, and stained with haematoxylin and eosin for pathological examination. Chimera formation iPSCs were microinjected into ICR host blastocysts and transferred into 2.5-day post-coitum ICR pseudopregnant recipient females. Chimerism was ascertained after birth by the appearance of black coat colour (from iPSCs) in white host pups. Western blot Cell extracts were prepared, resolved on gels, transferred to nitrocellulose and hybridized using antibodies against PUMA (1:1,000; Abcam, Cambridge, MA), p53 (1:1,000; Santa Cruz, Santa Cruz, CA), p21 (1:500; Santa Cruz, Santa Cruz, CA) and β-actin (1:500; Santa Cruz, Santa Cruz, CA). Images of full blots are provided in Supplementary Fig. S8 . Immunofluorescence Mouse iPSCs were cultured on a feeder layer in 12-well plate for 2–3 days until the colonies were formed. The cells were then fixed with 4% paraformaldehyde for 15 min, permeabilized with 0.1% Triton X-100 in PBS for 15 min and blocked with 5% BSA in PBS for 1 h at room temperature. After incubation with antibodies against mouse Oct4, Sox2, and Nanog (1:100 diluted in PBS containing 4% BSA, Santa Cruz, Santa Cruz, CA) overnight at 4 °C, cells were washed with PBS and incubated with secondary antibodies conjugated with Alexa 488 or Alexa 555 (1:1,000 diluted in PBS containing 4% BSA, Molecular Probes, Carlsbad, CA). For antibody staining of the cell surface protein, SSEA1 (1:500; R&D, Minneapolis, MN), the permeabilization step was not necessary. Apoptosis assay After transduction, the cells in the process of being reprogrammed were collected at days 1, 4, 8 and 12 after they were switched to ES culture medium. Untreated MEFs were used as controls. The cells were stained with the FITC Annexin V Apoptosis Detection Kit II (R&D, Minneapolis, MN) and propidium iodide (Sigma, St Louis, MO) according to the manufacturer’s recommendations and analyzed by flow cytometry with untreated MEFs as controls. To confirm the results, samples were subjected to TdT-mediated dUTP-biotin nick end labelling (TUNEL) testing to detect apoptosis by using the In Situ Cell Death Detection Kit (Roche, Branchburg, NJ). Detection of DNA double-strand breaks The cell at reprogramming day 4 and iPSC colonies at reprogramming day 12 were picked, digested with 0.5% trypsin and cytospun onto slides. The slides were then fixed with 2% paraformaldehyde for 15 min, permeabilized with 0.1% Triton X-100 in PBS and blocked with 5% BSA in PBS for 1 h at room temperature. The slides were incubated with mouse monoclonal antibodies against γ-H2AX (1:150 in PBS containing 2% BSA, Trevigen, Gaithersburg, MD) overnight at 4 °C and then secondary antibodies conjugated with Alexa 488 (1:200, Molecular Probes, Carlsbad, CA) for 1 h at room temperature. DAPI was used for nuclear staining. Images were produced with a confocal microscope (Leica, Buffalo Grove, IL) at × 600 magnification and analyzed for the number of γ-H2AX foci/nuclei. Karyotyping to assess chromosomal instability Briefly, cells were harvested following a 1-h treatment with 0.01 μg ml −1 Colcemid (Irvine Scientific, Santa Ana, CA) and ethidium bromide 1 μg ml −1 , hypotonic KCl (0.075 M) treatment for 30 min, followed by fixation and washes in 3:1 acetone-free methanol: glacial acetic acid. Slides for karyotype analyses were then prepared. GTG banding of the slides was performed by aging the slides overnight at 60 °C, followed by treating with EnZar-T trypsin (40 × ; 0.1 ml in 50 ml Hanks Balanced Salt Solution) for 45 s, 5% FBS in Hanks Balanced Salt Solution for 1 min, 15% Giemsa Stain in Gurr’s Buffer for 3 min. Slides were rinsed with tap water and air-dried. Microscopy was carried out using Olympus BX50 and Olympus BX61 bright field microscopes and the Genus Cytovision imaging system (Leica Microsystems, San Jose, CA). Twenty GTG-banded metaphase cells were studied from each of the four genotypes of MEFs and iPSCs. Chromosomal instability analysis included assessment of both numerical and structural chromosomal variability. Numerical changes refer to gain or loss of whole chromosomes. Structural abnormalities result from chromosomal breaks, detected by the presence of chromosome deletions, translocations, inversions, additional chromatin material of unknown origin and/or unidentifiable marker chromosomes. Anaphase and interphase bridges analysis We collected all kinds of genotypes of cells at reprogramming day 12 and MEF cells at passage 3 and reseeded them onto 22 × 22 mm glass coverslips with ~50,000 cells per coverslip. Cells were allowed to adhere and proliferate for 16 h prior to fixation and washing in cold acetone-free methanol. Coverslips were air-dried and stained with DAPI (40 μg ml −1 ) for 5 min followed by a rinse in ddH 2 0, air-dried again and mounted onto a microscope slide using antifade. Microscopy was carried out using an Olympus BX61 epifluorescence microscope and the Genus Cytovision imaging system (Leica Microsystems, San Jose, CA). Cell cycle and proliferation analysis Cell cycle and proliferation analysis assays were performed using Click-iT EdU Assay Kits. We selected pacific blue to show the EDU and 7-AAD to stain the DNA. The flow cytometry data were analyzed by Syan software. Statistical analysis Data represent means±s.e. Statistical analysis was performed using GraphPad Prism version 5.00 for Windows (GraphPad Software Inc., San Diego, CA, USA). Statistical significance was tested using the one-way ANOVA with Newman–Keuls post-test or a paired two-way Student’s t- test. P -values <0.05 were considered significant. How to cite this article: Li, Y. et al. The p53-PUMA axis suppresses iPSC generation. Nat. Commun. 4:2174 doi: 10.1038/ncomms3174 (2013).